The towering orogeny of New Guinea as a trigger for arthropod megadiversity Early studies on Melanesian mountain systems provided insights for fundamental evolutionary and ecological concepts. These island-like systems are thought to provide opportunities in the form of newly formed, competition-free niches. Here we show that a hyperdiverse radiation of freshwater arthropods originated in the emerging central New Guinea orogen, out of Australia, about 10 million years ago. Further diversification was mainly allopatric, with repeated more recent colonization of lowlands as they emerged in the form of colliding oceanic island arcs, continental fragments and the Papuan Peninsula, as well as recolonization of the central orogen. We unveil a constant and ongoing process of lineage accumulation while the carrying capacity of the island is about to be reached, suggesting that lineage diversification speed now exceeds that of landmass/new ecological opportunity formation. Therefore, the central orogeny of New Guinea acts as a motor of diversification for the entire region. Tropical mountains are highly diverse natural laboratories that provide an ideal setting for the study of macroevolutionary and ecological interactions during lineage diversification [1] , [2] . The tropical island of New Guinea in particular is exceedingly diverse [3] , and naturalists ever since Wallace [4] have used the island as a natural laboratory to study the evolution of species and communities [5] , [6] , [7] . The second largest island on Earth, New Guinea (>800,000 km 2 ), is situated in the tropics but contains an extraordinary diversity of climate zones and landforms. These range from lowland plains with a seasonal climate to alpine zones with permanent ice on high peaks (>4,700 m above sea level). The island contains many mountain ranges and some of the world’s last remaining tropical wilderness. Remarkably, most of this landmass was formed in the past 5 million years (Myr), resulting from major mountain building and what is arguably the world’s most complex geotectonic history [8] , further modified by extensive volcanism and glaciations [9] . Before 5 million years ago (Ma), and for much of the Cenozoic, the New Guinea region is thought to have been composed of many islands of varying geological origin ( Fig. 1 ). This archipelago structure played an important role in the local radiation of rainbow fishes [10] and in the global evolution of a major group of songbirds [11] , both c . 50–20 Ma. Speciation events resulting from island arc collisions and orogenies have been identified as key factors explaining the high biodiversity in Melanesia and in New Guinea in particular (general [3] , Aves [6] , Chelonii [12] , Odonata [13] , Hemiptera [14] , Heteroptera [15] ). 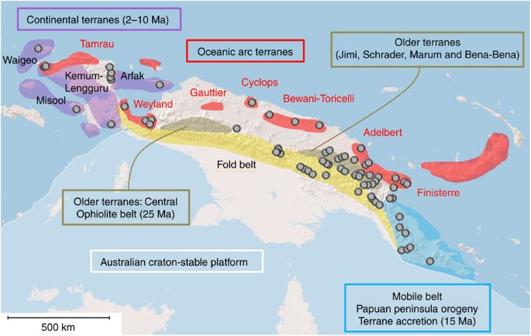Figure 1: Map of present-day New Guinea with major tectonic features and collecting localities for sequencedExocelinaspecimens. Filled circles indicate localities from which at least one specimen ofExocelinawas collected. Purple shading indicates continental terranes, red indicates oceanic arc terranes, brown indicates old terranes, and bright blue and yellow areas indicate the mobile and fold belts, respectively. The wide white area represents the Australian craton-stable platform. Figure 1: Map of present-day New Guinea with major tectonic features and collecting localities for sequenced Exocelina specimens. Filled circles indicate localities from which at least one specimen of Exocelina was collected. Purple shading indicates continental terranes, red indicates oceanic arc terranes, brown indicates old terranes, and bright blue and yellow areas indicate the mobile and fold belts, respectively. The wide white area represents the Australian craton-stable platform. Full size image Increasingly detailed paleotectonic data and more extensive, species-level molecular phylogenies provide the means to test different spatio-temporal and ecological scenarios for the rise and diversification of New Guinea biodiversity. The general approach has been used for studies of birds [10] , [16] , [17] , [18] , fishes [10] and mammals [19] , [20] , [21] , [22] , [23] . Results suggest that species-level diversification within New Guinea has been recent (<5 Ma), corroborating geological evidence that dates substantial landmass formation to <10 Ma [24] , [25] . Lowland vertebrate taxa tend to exhibit north–south divergence on either side of the predominant east–west cordillera [10] , [16] , [26] . Montane taxa more commonly exhibit east–west splits, thought to result from more local allopatric speciation among drainages along the cordillera [27] . Although New Guinea remains a region where comparatively few geological studies have been carried out (due to its difficult terrain, remote location and climate), plate tectonic models for the development of New Guinea have been proposed recently based on the evidence available. A model proposed by van Ufford and Cloos [28] suggested that an underthrusting of the Australian continent beneath an Inner Melanesian arc resulted in an orogeny restricted to eastern New Guinea c . 35–30 Ma. A later orogeny (from 15 Ma in the west to 3 Ma in the east) then gave rise to the Central Range at its present elevation c . 5 Ma. Biogeographically, this model [28] would suggest the Papuan Peninsula in eastern New Guinea to be an area of early lineage diversification [13] , with successive lineages arising along the central range out of the Papuan Peninsula. In contrast, Hall [29] , and Hill and Hall [30] proposed that convergence between the Pacific and Australian plates c . 5 Ma formed a fold-and-thrust belt and led to rapid rise of the central ranges that continues today. This model implies that New Guinea was largely submerged until the Early Pliocene and that formation of the present large emergent area occurred in the last 5 Ma [24] . Under this model, the expected biogeographic pattern would be rather divergent from the van Ufford and Cloos model [28] with an expected early diversification on the fold and thrust belts corresponding to present-day central orogen, followed by colonization of surrounding areas such as the oceanic terranes drifting from the North, the Bird’s Head and the Papuan Peninsula. Despite their overwhelming contribution to animal diversity, studies of invertebrate diversification on New Guinea remain in their infancy (but seerefs 7 , 31 ). In contrast to vertebrate diversification in the recent past on the landmass, invertebrate speciation on ancient island arcs is thought to be important in shaping extant species richness and distribution patterns [13] , [14] even though alternative hypotheses implying Quaternary diversification on the island exist [7] . Nonetheless, the macroevolutionary and macroecological drivers of their diversification remain little understood, and species-level patterns have yet to be tested in a phylogenetic framework. Here we combine dense sampling of a single lineage of predaceous diving beetles (Dytiscidae, Exocelina ) with molecular phylogenetics and sophisticated biogeographical and diversification analyses to test alternative geological scenarios and examine how extensive environmental change and very recent formation of most New Guinea terrestrial habitats have interacted to promote lineage diversification. We reconstruct a dated species-level phylogeny to analyse ancestral states and rates of lineage diversification and use this to test alternative hypotheses of (i) older island arc evolution [14] , [15] and (ii) early mountain building in the present Papuan Peninsula [13] of eastern New Guinea versus (iii) evolution and diversification in a more recent central orogen [29] , [30] with subsequent colonization of other areas in the New Guinea region. Our findings indicate that lineage diversification was comparatively recent, driven by the formation and subsequent modification of the central highlands, and that all other areas of New Guinea were colonized out of that region. Rather than being unidirectional, diversification into lower altitudes was reversed several times and included secondary highland radiation. We conclude that lineage diversification is a recent, complex, and dynamic process, in our case not closely linked to terrane movement as has been largely assumed. Molecular phylogenetics The final concatenated alignment comprised 4,299 bps sequenced for 94 New Guinean Exocelina diving beetle species: 1,593 bps of mitochondrial cytochrome c oxidase I ( cox1 ), cytochrome c oxidase II ( cox2 ) and cytochrome b ( cob ) gene fragments, in addition to 2,706 bps of the nuclear histone 3 ( H3 ), histone 4 ( H4 ), 18S rRNA ( 18S ), Carbomoylphosphate synthase ( CAD ) and Alpha-Spectrin ( Asp ) gene fragments. The Bayesian phylogenetic analysis based on the combined data set and the best-fitting partitioning scheme ( Tables 1 and 2 ) yielded a highly resolved and strongly supported tree highly compatible with the tree generated in the RAxML analysis ( Supplementary Figs 1 and 2 ). Table 1 Partitioning schemes for the Bayesian inference analyses. 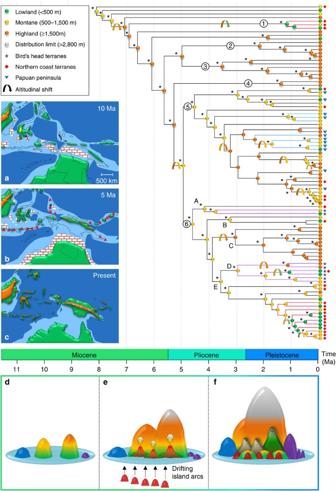Figure 2: Dated Bayesian phylogeny of the New GuineanExocelinaradiation and paleotectonic evolution of the New Guinean archipelago. A time-scale is indicated spanning the full evolutionary history of the group. Asterisks above the nodes indicate strong support (PP≥0.95) for the reconstruction of the ancestral altitude state. Pastilles code for vertical distribution according to legend; purple stars=distribution on continental Bird’s Head terranes; red diamonds=north coast terranes; blue triangles=Papuan Peninsula. Coloured branches indicate the reconstruction of the ancestral horizontal distribution state (black branches=central orogen). Panelsa–con the left side show maps of the distribution of land and sea at respectively 10 Ma, 5 Ma and at present after ref.21(green, land; dark blue, deep sea; lighter blue, shallow sea; red white brick, calcareous plateaus possibly exposed at times; orange, highland; grey, high altitude above 2,800 m). All maps are at the same scale indicated ina. Below is a schematic summary in a South-to-North orientation of major tectonic processes from proto- to present day New Guinea. Panelsd–fhighlight the orogenic dynamics that took place during the evolution of theExocelinaradiation respectively between 12–8 Ma, 8–4 Ma and 4–0 Ma. Far right in purple: drifting and colliding continental Bird’s Head terranes; front in red: north coast terranes; central orogen with altitudinal zones colour codes as on the tree, Papuan Peninsula in blue at the far left. Numbers and letters in the tree refer to the major clades and subclades of the radiation. Full size table Table 2 Best-fit partitioning strategies for the BI analyses with Bayes factors (BF) estimates. Full size table We recover a succession of branching events at the deepest level in the tree and six major clades in a more derived position ( Fig. 2 ), for example, clade 6, corresponding to the Exocelina ekari group [32] . Sequence divergence was low, for example, in cox1 the smallest interspecific uncorrected P distance was only 1.7% (s.d., 1.48) and the mean interspecific distance was 5.82%. Overall, interspecific divergence ranged from 0–9.2%. This was reflected in a shallow branching pattern at the tips as well as species clustering, which even at 1% threshold only recovered 69 clusters instead of the expected 94 due to lumping of taxonomic species. These results pinpoint that several species diverge by <1%: the parapatric E. atowaso + E. astrophallus by (0.67%, despite divergent male genital morphology), the allopatric E. wondiwoiensis + E. irianensis (0.13%, male genital similar) and the sympatric (not yet found syntopic) E. weylandensis + E. soppi (0.14%, male genital moderately divergent) [32] . Figure 2: Dated Bayesian phylogeny of the New Guinean Exocelina radiation and paleotectonic evolution of the New Guinean archipelago. A time-scale is indicated spanning the full evolutionary history of the group. Asterisks above the nodes indicate strong support (PP≥0.95) for the reconstruction of the ancestral altitude state. Pastilles code for vertical distribution according to legend; purple stars=distribution on continental Bird’s Head terranes; red diamonds=north coast terranes; blue triangles=Papuan Peninsula. Coloured branches indicate the reconstruction of the ancestral horizontal distribution state (black branches=central orogen). Panels a – c on the left side show maps of the distribution of land and sea at respectively 10 Ma, 5 Ma and at present after ref. 21 (green, land; dark blue, deep sea; lighter blue, shallow sea; red white brick, calcareous plateaus possibly exposed at times; orange, highland; grey, high altitude above 2,800 m). All maps are at the same scale indicated in a . Below is a schematic summary in a South-to-North orientation of major tectonic processes from proto- to present day New Guinea. Panels d – f highlight the orogenic dynamics that took place during the evolution of the Exocelina radiation respectively between 12–8 Ma, 8–4 Ma and 4–0 Ma. Far right in purple: drifting and colliding continental Bird’s Head terranes; front in red: north coast terranes; central orogen with altitudinal zones colour codes as on the tree, Papuan Peninsula in blue at the far left. Numbers and letters in the tree refer to the major clades and subclades of the radiation. Full size image Divergence times and diversification The chronogram derived from the relaxed molecular clock analyses of cox1 suggested a colonization of New Guinea occurring during the late Miocene (median age 8.2 Ma, 95% HPD 6.2–10.7 Ma; Fig. 2 and Supplementary Fig. 3 ) with most of the branching events occurring in the Plio-Pleistocene (5.3–0 Ma). The TreePar diversity-dependent analyses carried out on the chronogram support a birth–death model with no diversification rate shift during the evolution of the radiation. 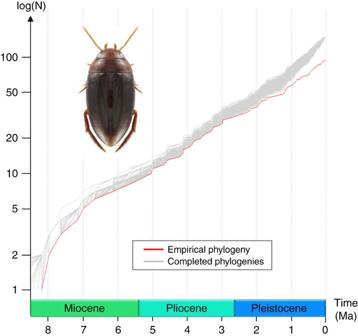Figure 3: LTT plots of the New GuineanExocelinaradiation. A time-scale is indicated spanning the full evolutionary history of the group. The vertical axis shows the number of species in logarithmic scale. The LTT plots of the New GuineanExocelina(E. unipois presented) have been generated using the BEAST incomplete phylogeny (red line) and 1,000 simulated complete phylogenies (grey lines) to illustrate the constant diversification of the radiation fostered by the orogeny of the island. This model corresponds to a pattern of constant accumulation of lineages through time with a rather high rate of diversification ( r =0.3950) ( Table 3 ). The density-dependent analyses indicate that the maximum carrying capacity K is about to be reached (150/169) and that therefore the radiation will soon attain equilibrium. The lineage-through-time (LTT) plots inferred using either the BEAST incomplete phylogeny or 1,000 simulated phylogenies accounting for missing taxon sampling highlight the pattern of constant accumulation of Exocelina lineages during the evolution of the radiation ( Fig. 3 ). Table 3 Results from the TreePar analyses conducted on the BEAST chronogram. Full size table Figure 3: LTT plots of the New Guinean Exocelina radiation. A time-scale is indicated spanning the full evolutionary history of the group. The vertical axis shows the number of species in logarithmic scale. The LTT plots of the New Guinean Exocelina ( E. unipo is presented) have been generated using the BEAST incomplete phylogeny (red line) and 1,000 simulated complete phylogenies (grey lines) to illustrate the constant diversification of the radiation fostered by the orogeny of the island. Full size image Ancestral state reconstructions For the altitudinal species distribution, the first three nodes of the tree backbone had strong support (posterior probability (PP) ≥0.95) for the ‘≥500 m’ state, followed by ‘≥1,500 m’ at the 4th node. The earliest lineages in the evolution of the radiation, including clade 1, have independently colonized lowland and highland parts of the island from an initial montane zone during the past 8 Myr. Clades 2 and 3 contain species from the uppermost distributional limits, 2,000–2,800 m. Lower altitude colonization is a more recent event, independently occurring in clade 5 and with significant diversification in clade 6. The results of the ancestral character state optimization for the horizontal origin trait recovered a central orogen origin with strong support (PP=1.0). This character state also was recovered for most of the internal nodes with strong support (PP≥0.95). Multiple shifts from central orogen to north coast range terranes (NCR) from the early Pleistocene were recovered with strong support (PP=1.0), although the ancient lineage E. undescribed species MB1530 now occurs in the NCR. The colonization of the Bird’s Head terranes (BHT) had a comparable timing in clade 6D, with subsequent radiation; one species ( E. undescribed species MB1269, clade 6A) colonized the BHT earlier. Topological patterns congruent with speciation along an island arc were only recovered for the three NCR species in clade 1 ( Fig. 2 ), with one species each occurring in the Cyclops, Bewani and Adelbert Mountains ( Fig. 1 ). Their diversification is here inferred from the Pleistocene. The supposedly very old Papuan Peninsular orogen was colonized several times from western parts of the central highlands ( Fig. 2 ). Competitive exclusion On the basis of our preliminary co-occurrence matrix, we found that up to five species were sampled from the same habitat (puddle or stream segment). Relative abundances appeared to differ although precise quantification was outside the scope of our collecting regime. In general, syntopic species were not closely related. Only In the E. ekari clade 6E did we find several closely related species syntopically, for example, E. weylandensis , E. soppi , E. kakapupu and E. utowaensis ( Supplementary Fig. 4 ). Local diversity appears mostly to result from repeated colonization by different lineages. An example is the syntopic occurrence of highland species from the older clade 2 with species of clade 6C that have recently colonized the highlands from lower elevations. New Guinea is situated at the convergent boundary of the Australian and Pacific plates. Present-day New Guinea is a geologically young landmass of heterogeneous origin, composed of many terranes [33] , including obducted ophiolites, accreted oceanic island arcs, continental slivers and the Australian continental margin [8] , [24] . In general terms, southern New Guinea and several sections of the western New Guinea (for example, the Bird’s Head peninsula) are, or have been, formed from parts of the Australian plate ( Fig. 1 ). The spine of New Guinea is a 1,300-km-long and up to 150-km-wide central highland chain. It includes a major fold-and-thrust belt in the central range that represents the deformed passive margin of the Australian continent, to the north of which are ophiolite belts (oceanic or arc lithosphere displaced during island arc–continent collision) and accreted island arc terranes. The ophiolites and arc terranes have been described as part of a mobile belt [30] , [34] in which there was significant deformation during the Neogene since ~25 Ma. Early studies interpreted New Guinea in terms of terranes [33] , [35] , which are fault-bounded crustal fragments each with its own geological character, and suggested that at least 32 terranes had been added to the Australian margin in a series of collisions linked to subduction during the Cenozoic. A tentative plate tectonic model based on this terrane concept was outlined by Struckmeyer et al. [36] Later models [28] , [29] , [30] , [34] viewed New Guinea development in a more comprehensive plate tectonic framework, although there remain considerable differences between different models in terms of timing, events and inferred plate reconstructions. van Ufford and Cloos [28] proposed a model which included two intra-oceanic arc systems north of New Guinea subducting discontinuously to the north and south from the Eocene to Middle Miocene with numerous small subduction zones developed since. In their model there is no role for the Philippine Sea plate and they interpreted several small plates between the Pacific and Australian plates. They suggested that at 35–30 Ma underthrusting of the Australian continent beneath their Inner Melanesian arc resulted in a peninsular orogeny. This orogeny was restricted to eastern New Guinea and initiated uplift and emergence of the Papuan Peninsula. Much later, the Central Range orogeny commenced 15 Ma in the west and up to 3 Ma later in the east, and was proposed to result from contractional thickening of passive margin strata and underthrusting of Australian continental basement. According to this model deformation began at the distal northern edge of the Australian passive margin where sediment cover was removed from oceanic or transitional crust, and collisional orogenesis involving continental crystalline basement began at 8 Ma. van Ufford and Cloos [28] observed a dramatic change in the coarseness and extent of clastic sediments, which they attribute to the rise of the Central Range to its present elevation at about 5 Ma. Hall [29] , and Hill and Hall [30] proposed a very different model. They suggested there was subduction during the Paleogene beneath a Philippines–Halmahera–Caroline intra-oceanic arc system after the Australian plate began to move rapidly northwards in the Eocene. Collision with the Philippines–Caroline arc commenced in the Late Oligocene at ~25 Ma. This caused a change to sinistral oblique convergence with the Philippine Sea and Pacific–Caroline Plates, which resulted in Paleogene arc fragments being displaced westwards along the New Guinea margin and sliced into many smaller terranes. The New Guinea Mobile Belt thus represents the complex Neogene strike-slip zone to the north of the Australian passive margin with over 1,000 km sinistral displacement that has alternated between extension and compression. It is in this region that there were possibly small emergent areas during the Miocene. A change in plate motions at about 5 Ma initiated convergence between the Pacific and Australian plates and caused the formation of the fold and thrust belt and rapid rise of the central ranges that continues today. This model implies that New Guinea was largely submerged, except possibly for parts of the New Guinea Mobile Belt, until the Early Pliocene and that the formation of the present large emergent area occurred in the last 5 Ma [24] , as mentioned above. In the space of this paper it is not possible to discuss the reasoning and conclusions of these different geological models for New Guinea except to agree that ‘…the age, number and plate kinematics of the events that formed the island are vigorously argued’ [28] . Nonetheless, despite significant differences in interpretation of events and plate tectonic reconstruction, the two models [28] , [29] , [30] have some features in common as far as the distribution of land is concerned. From the Oligocene until the Late Miocene there was likely to have been only small areas of land at the Pacific margin north of New Guinea. Disconnected islands may have formed where there were volcanic arcs, at local uplifts near to plate boundaries and in the Mobile Belt. There was shelf carbonate deposition along much of northern Australian margin in what are now the New Guinea ranges. From the Late Miocene there is evidence of increased siliciclastic sediment input, indicating erosion of land areas, and both models infer that massive and rapid uplift from 5 Ma formed the highest summits (3,000–5,000 m), accompanied by steady widening of the central ranges. Since 5 Ma, strike-slip movements in the northern part of New Guinea have also contributed to the current topography. Although precise timing is uncertain, it is clear that many parts of northern New Guinea, from the Bird’s Head to New Britain, emerged above sea level in this period [24] , [25] , [28] , [30] . The major differences between the two models for biogeographers are that the first model [28] would suggest the Papuan Peninsula as an area of early lineage diversification and a successive phylogenetic tree branching pattern along the central range in an east–west direction, whereas the alternative [29] , [30] implies much younger colonization and diversification, centred on the Central Range. Our results, based on the most extensive molecular phylogenetic and biogeographic species-level analysis for any New Guinean taxon to date, suggest a recent origin of New Guinean Exocelina during the late Miocene (~8.2 Ma) and a constant process of lineage diversification. The ongoing diversification suggests species have continuously colonized the plentiful, newly formed, biologically empty habitat. However, as highlighted by the calculated carrying capacity of the radiation, the diversification process might experience a slowdown in the next million years, corresponding to a saturation of ecological niches and habitat on the island. This pattern would imply that the rate of diversification will eventually exceed the pace of ecological opportunity formation fostered by the ongoing orogeny of the island. The ancestral character state reconstructions revealed two important ancestral traits: an early occurrence at montane elevation, and an origin in the central orogen. In a geologically dynamic landscape like New Guinea, it is however difficult to infer ancestral altitudinal preference, because we have data only from present-day distributions. Ancestral New Guinea Exocelina might have colonized lower altitudes, diversified and undergone passive uplift to the high altitudes. They may also have colonized higher altitudes and migrated into lower areas as compensation for uplift into zones with colder temperatures. We suggest a complex mixture of both scenarios, as we uncovered several altitudinal shifts in our analysis. Ancestral Australian Exocelina are lowland species [37] , which suggests lowlands may be the ancestral New Guinea habitat. During mountain uplift along the northern margin of the Australian plate, an initial colonization out of Australia [37] would have reached emerging islands that might have had some elevation already. At that stage, the emerging orogen would have been an insular setting supporting lineage diversification, analogous to the initial branching found in rainbow fishes [10] . Strong landscape changes during the uplift as well as significant amounts of volcanism during the late Neogene followed by Quaternary climate change [9] likely shifted environmental conditions. These changes would have further promoted the isolation of populations and fuelled lineage diversification [7] , [12] , [14] . The extremely structured central highland chain itself, with ongoing formation of rich aquatic resources in particular during the formation of extensive foothill chains, provided the setting for random colonization of new areas followed by isolation and speciation in remote valleys or mountain blocks [38] . Interestingly, New Guinean Exocelina are almost exclusively associated to running waters, and there is evidence that species in such habitats are weak dispersers. This trait has been suggested to enhance allopatric speciation and micro-endemism in diving beetles [39] , and could therefore represent one of the underlying mechanisms fostering this astonishing radiation. More generally, tropical species are thought to be adapted to rather narrow climatic conditions because they do not experience seasons [40] . Colonization of new vertical bands might therefore be rare enough to support isolation. Others have proposed that the present-day diversity of the New Guinea fauna is the product of ancient geological processes and landmass collisions. Instead, we found that this was not the case. The terranes of the oceanic South Caroline arc that formed much of the NCR, and the continental terranes that formed the Bird’s Head and satellite islands, have been colonized from the central orogen after these different landmasses attained some proximity or had docked already. Previous hypotheses assigned a central role to these terranes in the diversification of diverse arthropod lineages on drifting island arcs. The biota was proposed to have reached island arcs while adrift in the Pacific, with subsequent diversification along the island arc, on islands remote from each other and from the rest of the emerging New Guinea [15] (also refer to the ‘Discussion’ in ref. 12 ). Closely related species would have reached closer geographic proximity only after terrane collision [15] . Analytically, this would predict (1) a greater age of the species on fully insular arcs far from the rising orogen, 40–10 Ma, and (2) a tree topology with no closely related species in other parts on present day New Guinea. It also implies that islands arcs did indeed provide terrestrial ecosystems over a long period of time, which is far from being unambiguously proven (ref. 24 , page 116). Our results provide strong evidence for an alternative and more complex scenario, namely that recent environmental change in the central highlands has been the primary driver of diversification in New Guinea. The evidence from tree topology, ancestral range reconstruction and lineage ages do not support the hypothesis of an older, island-arc evolution on the NCR and Bird’s Head terranes [14] , [15] . Instead, the data indicate repeated colonization in the recent past. Present-day alpha-diversity thus appears more related to colonization events than to local diversification in a given terrane. The pattern expected from an older, island-arc scenario was seen only in clade 1, where single species occurred in each of the Cyclops, Bewani and Adelbert Mountains. While the clade was comparatively old, the species in each mountain range appear to have arisen in the last 2 Myr. This suggests recent allopatric speciation along the north coast as opposed to on ancient islands adrift. The relative isolation of the Bird’s Head [12] was also suggested by our findings. There have been only two colonization of Exocelina , both of which appear to be recent ( Fig. 1 ). This does not lend support to hypotheses of evolution on terranes adrift. The lack of colonization of the Bird’s Head may be attributed to a lack of suitable stream habitats in the karstic geology of the Lengguru area that connects the Bird’s Head with mainland New Guinea. The sister species to all other New Guinea Exocelina occurred in the Adelbert Mountains of the NCR, but its origin was the central orogen according to the ancestral range reconstructions. Related species occur along the central orogen as well. The hypotheses of early mountain building in eastern New Guinea were also not supported by our biological data. Exocelina diving beetles have colonized the Papuan Peninsula up to the Herzog Mountains out of the central orogen at least six times in comparatively recent time. Distribution at high altitude in clades 2 and 3 was usually allopatric, related species occurring on different mountains. Thus, Exocelina do not exhibit a pattern described by Diamond [6] , who identified (ecological) montane speciation in the absence of ecotones as a source of New Guinea bird diversity, where sister species occupy sharply delineated altitudinal zones on the same mountain. Allopatry appears to be the main mechanism in Exocelina, in general along more or less the same altitudinal zone as far as can be seen from our sampling. This differs from speciation patterns observed in the few other studies of running water organisms, where there is evidence that speciation may follow the river course longitudinally in peripatric speciation. Spatial patterns of speciation in running waters have interested ecologists since Illies [41] , who suggested that warm-adapted lineages of aquatic insects arose from cold-adapted ones, with evolution within river systems progressing downstream. Statzner and Dolédec [42] found empirical evidence for this based on the distribution of ecological traits and phylogenetic relationships among French Hydropsyche (Trichoptera) species. They suggested a headwater ancestor with primarily downstream evolution of the clade. In contrast, Malagasy mayflies (Ephemeroptera) appear to have diversified from lowland ancestors to colder and faster-flowing upstream sections [43] . The syntopic or near-syntopic presence of closely related Exocelina species in the Weyland area ( Fig. 2 , clade 6E; Supplementary Fig. 4 ) suggests that peripatric speciation mechanisms may also contribute to the observed species richness, but the consistency of the pattern remains to be tested using denser longitudinal sampling. There are no detailed ecological studies of Exocelina species in New Guinea. We observed that the relatively recent clade 6 includes many lowland species adapted to peripheral habitats along fast-flowing streams. Species in clades 2 and 3 live in habitats with slower flows that are similar to the habitat of the older lineages of Exocelina that occur in Australia. This suggests diversification into new, more extreme habitats, with the result that more emerging habitats are being utilized. Here, too, denser sampling is needed to further study mechanisms at work, that is, possible niche segregation and different abundances among sites. In summary, our extensive biological data set implicates recent diversification and repeated colonization of sites by distantly related lineages as the primary drivers of the diversity patterns found in New Guinea Exocelina. Despite the clear biological results, a number of questions remain. In terms of geology, the origin of the Weyland and Wandammen regions remain unresolved. The extent and configuration of land available for colonization is still uncertain, but the general setting summarized above provides the framework for investigations of the biological evolution of New Guinea. Data from biologists and a large selection of organisms could potentially inform geologists about land configurations in the past, supporting a truly integrative science. Taxon sampling and phylogenetic analyses Using standard protocols ( Supplementary Table 1 ) we obtained sequences from 94 in-group species from across New Guinea and representing all known morphological groups ( Supplementary Table 2 ) [32] . Three species of Exocelina from Australia and New Caledonia were included as close outgroups as well as two representatives of the subfamily (Copelatinae); Copelatus irregularis , Lacconectus peguensis and Thermonectus sp (Dytiscinae) in order to root the tree. We sequenced fragments of mitochondrial cox1 (735 bp used in our alignment), cox2 (552 bp) and cob (306 bp), as well as nuclear H3 (318 bp), H4 (198 bp), 18S (570 bp), CAD (828 bp) and Asp (792 bp). Sequences were edited using Geneious R6 (Biomatters, http://www.geneious.com ), aligned with Muscle [44] and codon positions were determined using Mesquite 2.75 ( http://mesquiteproject.org ). We used Bayesian inference (BI) and maximum likelihood (ML) on the concatenated data set containing one specimen per species and seven different partitioning strategies ( Table 1 ) to account for expected differences in sequence evolution in different genes. The best model for each partition was selected under jModelTest 2.1.3 (ref. 45 ), using the corrected Akaike information criterion (AICc) ( Supplementary Table 3 ). An additional scheme was tested based on the partitions selected in PartitionFinder 1.1.1 (ref. 46 ) under the AICc ( Table 1 ). The BI analyses were run in MrBayes 3.2 (ref. 47 ) with two independent runs consisting of eight Metropolis-coupled Markov Chains Monte Carlo (MCMC, one cold and seven incrementally heated) running for 50 million generations and sampling every 1,000 cycles. The split-frequencies and log-likelihood curves were investigated before applying a conservative burn-in of 25%, and the remaining topologies were used to generate a 50% majority rule consensus tree. The best strategy of partitioning was selected afterwards based on Bayes factors (BF) [48] and effective sample size (ESS) criteria approximated under Tracer 1.5 (ref. 49 ). BF tests were based on marginal likelihoods calculated using stepping-stone sampling to account for harmonic mean unsuitability to deliver unbiased estimates [50] , [51] . BF values superior to 10 were considered good indicators of a significantly better partitioning scheme over another, and ESS values greater than 500 indicative of a good convergence of the runs [52] . The ML analyses were carried out with the best model found in BI under RAxML [53] . We performed 5,000 ‘thorough bootstrap’ replicates (BS) to investigate the level of support for each node. Calculated PP values ≥0.95 and BS values ≥70 were considered to indicate strongly supported nodes [54] , [55] . Estimation of divergence times In order to calibrate the topology and since the fossil record is scarce for diving beetles, we used the information of three recent publications on Coleoptera in which a divergence rate for the same cytochrome c oxidase subunit 1 fragment used in this study was calculated, that is on dytiscid beetles [56] (mean rate=0.0195 substitutions per site per million years per lineage, subs/s/Myr/l), on tenebrionid beetles [57] (mean rate=0.0177 subs/s/Myr/l) and on carabid beetles [58] (mean rate=0.0145 subs/s/Myr/l). We set the ucld.mean with a normal distribution encompassing the three mean rates recovered in these studies (0.0145–0.0195 subs/s/Myr/l). To test the putative clockwise evolution of the matrix, we used PAUP* [59] and calculated likelihood with and without a strict molecular clock. The likelihood ratio test conducted under the same software resulted in a P value<0.001, implying that the strict molecular clock assumption was not statistically supported. Therefore, we used a relaxed clock model allowing rate variation among lineages. We carried out the analyses using the BEAST 1.7.4 (ref. 60 ) with the following non-default settings and priors: the Site Model was chosen according to the models of evolution used in the phylogenetic analyses, the Molecular Clock Model was set to an estimated Relaxed Clock: Uncorrelated Lognormal , the Tree Model to a Speciation: Birth Death Process and the MCMC parameters were fixed to 30 million generations with sampling every 1,000 generations and the first 10% discarded as burn-in. The best topology recovered from the BI phylogenetic reconstructions was fixed by manually editing the .xml file generated in BEAUTI 1.7.4 (ref. 60 ). Ancestral state reconstructions The ancestral state reconstructions were performed using the ‘ Traits’ and ‘ Sates’ options in the BEAST 1.7.4 (ref. 60 ) on the chronogram from which we pruned all outgroups. For the reconstruction of the ‘Altitude’ character, each species was assigned to one of the following categories: ‘Lower altitude <500 m’, which would capture species in lowland-foothill forest across the island, warmer climate and often faster-flowing streams on steep foothill slopes; ‘Montane 500–1,500 m’ as the lower montane zone leading towards the actual highlands, often fast flowing; and ‘Highland ≥1,500 m’, or mid montane zone, which contains the large intra-montane depressions of New Guinea up to the montane cloud forests. These bands are following altitudinal zonation and to some degree generalized due to regional differences in zonation [61] , [62] . For the ‘Horizontal distribution origin’ character, we use a generalized scheme, according to the two major island arcs or terrane systems that have formed distinct, clear cut geographic features of the island: the Bird’s Head Including the Satellite islands in the west and the NCR. Finally, the central mountain range as well as the inferred older terranes closely attached to it in the north, and which drop into lowlands, marking a comparably clear-cut transition towards the NCR. E. brahminensis and E. astrophallus occur in NCR as well as the basin between central range and NCR, and were assigned to NCR. E. cf. brahminensis was reported from the Herzog Mountains [32] , northern Papuan Peninsula, but we had no sequence data from that locality and decided to code our NCR specimens as NCR only. All analyses were run until the ESS of each parameter reached 500 and 25% of the samples were discarded as burn-in before generating the maximum credibility tree in TREEANNOTATOR 1.7.4 (ref. 60 ). Diversification analyses We assessed the diversification pattern of the Exocelina radiation using the ape [63] , TreePar [64] and TreeSim [65] packages for R and the BEAST chronogram from which we pruned all outgroups. We used the approach developed by Stadler [64] to estimate putative shifts in speciation and extinction rates in possibly incomplete phylogenies. We used the function ‘ bd.shifts.optim’ to estimate the ML speciation and extinction rates along with the possible shift times in the Exocelina radiation. As an input, the function requires the number of sampled taxa in the phylogeny as well as an estimation of the current species richness in the clade. The analyses were therefore run with the following settings: the taxon sampling was set to 94 species and the extant diversity to 150 species, start=0 and end=8 and grid=0.1 Myr for a fine-scale estimation of rate shifts. The best-fitting model was selected on the basis of likelihood ratio tests. We also used the method of Etienne et al. [66] implemented in TreePar to test for a potential saturation of Exocelina diversity on the island. Hence, we explored the effect of diversity on speciation and extinction rates. The function ‘ bd.densdep.optim ’ was used to fit this model with the following settings: discrete=TRUE, missing species acknowledged using ρ =94/150, the initial carrying capacity fixed to the extant diversity minK=150 and the maximum carrying capacity tested fixed as a default parameter to maxK=1.5 × minK=225. Finally, we constructed LTT plots to visualize diversification rate over time using ape [63] for the 94 species included in this study and TreeSim [65] to draw the LTT of 1,000 simulated topologies accounting for missing taxa under a constant rate model [67] . Bionomics Based on the sequenced specimens, as well as >3,000 additional specimens currently under taxonomic study, we compiled a preliminary survey of species composition per collecting locality. Most of our collecting localities only contain samples from one puddle or several small waterholes along one stream segment less than 200 m long. These data were used to evaluate the extent to which sister species or close relatives co-occur. Accession Codes : Sequences have been deposited in EMBL Protein Knowledgebase database under accession numbers HG974147 to HG974233 and HG973548 to HG973881 . How to cite this article: Toussaint, E. F. A. et al. The towering orogeny of New Guinea as a trigger for arthropod megadiversity. Nat. Commun. 5:4001 doi: 10.1038/ncomms5001 (2014).